Early Eocene fossils suggest that the mammalian order Perissodactyla originated in India Cambaytheres ( Cambaytherium , Nakusia and Kalitherium ) are recently discovered early Eocene placental mammals from the Indo–Pakistan region. They have been assigned to either Perissodactyla (the clade including horses, tapirs and rhinos, which is a member of the superorder Laurasiatheria) or Anthracobunidae, an obscure family that has been variously considered artiodactyls or perissodactyls, but most recently placed at the base of Proboscidea or of Tethytheria (Proboscidea+Sirenia, superorder Afrotheria). Here we report new dental, cranial and postcranial fossils of Cambaytherium , from the Cambay Shale Formation, Gujarat, India (~54.5 Myr). These fossils demonstrate that cambaytheres occupy a pivotal position as the sister taxon of Perissodactyla, thereby providing insight on the phylogenetic and biogeographic origin of Perissodactyla. The presence of the sister group of perissodactyls in western India near or before the time of collision suggests that Perissodactyla may have originated on the Indian Plate during its final drift toward Asia. Perissodactyla, Artiodactyla and Primates are extant mammalian orders that appeared abruptly at the beginning of the Eocene across the Holarctic continents [1] , with little indication of their source. The precise phylogenetic and biogeographic origin of these orders is one of the great conundrums of mammalian evolution. Perissodactyls, including extant horses, rhinoceroses and tapirs, were long held to be closely related to or derived from the Palaeocene–Eocene ‘condylarth’ (archaic ungulate) family Phenacodontidae [2] , although this relationship is now considered equivocal [3] , [4] , [5] . Recent analyses of molecular data [6] , [7] , [8] and combined morphological and molecular matrices [9] , [10] place Perissodactyla and Artiodactyla in Laurasiatheria, well separated from Afrotheria. Afrotheria includes Hyracoidea and Tethytheria, which were allied with Perissodactyla and Phenacodontidae to the exclusion of Artiodactyla in some earlier morphological studies [11] , [12] . Combined analyses of morphology and molecules have placed phenacodontids either with afrotheres [9] or at the base of Laurasiatheria [10] . While their role in perissodactyl origins is unclear, phenacodontids preserve a suite of ancestral features that provide useful comparisons when discussing perissodactyl origins. The geographic source of Perissodactyla is also unclear, although recent authors have favoured an Asian origin [3] , [13] . One scenario proposed that perissodactyls are among clades that may have originated from primitive eutherian stock on India during its northward drift [14] , but until recently no fossil evidence existed to test this hypothesis. Discovery over the last decade of very primitive primates, artiodactyls and cambaytheres in the early Eocene Cambay Shale Formation of Gujarat, India [15] , [16] , [17] , [18] , [19] —the oldest known vertebrate-bearing Cenozoic strata in India—confirms that India played a significant role in the earliest radiations of these Holarctic orders. Cambaytherium was originally described as a bunodont perissodactyl, comprised of multiple species [15] , [16] . A closely related cambaythere from Vastan mine, Kalitherium marinus , is based on a poorly preserved rostrum about 50% larger than that of Cambaytherium thewissi [15] . It is otherwise very similar to Cambaytherium and it, too, was placed in Perissodactyla. However, other taxa that can now be shown to be cambaytheres ( Nakusia shahrigensis [20] , Indobune vastanensis [17] ) were originally allocated to Anthracobunidae, a family most recently interpreted as either stem Tethytheria [21] or stem Proboscidea [11] , [20] , [22] , [23] , [24] . Anthracobunidae were previously considered either artiodactyls or perissodactyls [25] . Nakusia , from the early Eocene of Baluchistan, Pakistan, was based on a worn maxillary dentition that is almost indistinguishable from Cambaytherium and is surely closely related. Upper teeth from Vastan mine that are very similar to those of Nakusia , and also show close similarity to the anthracobunid Pilgrimella , were described as a new anthracobunid Indobune vastanensis [17] ; but based on the sample described here they are clearly the upper teeth of C. thewissi . Thus, all of these are closely related cambaytheres, although they have been interpreted as either perissodactyls (laurasiatheres) or anthracobunids (supposed afrotheres). Deciphering the true relationships of cambaytheres is essential to understanding the early radiation of these clades, and the new material reported here establishes their phylogenetic position with confidence. The vertebrate fossils from the Cambay Shale Formation are estimated to be about 54.5 Myr based on dinoflagellates [26] and stable isotope records [27] , [28] . They come mainly from small, thin lenses of carbonaceous shale, representing nearshore continental sediments, that occur 1–3 m above the lower of two major lignites (Lignite 2) present at Vastan and Mangrol mines [17] , [18] , [29] , [30] . The vertebrates are closely associated with plant fossils and amber indicating that they lived in or near a coastal tropical rainforest dominated by Dipterocarpaceae [31] . Three dinoflagellate species from the zone producing the vertebrates imply an age not older than 55 Myr; one species from about 12 m higher than the vertebrates has been interpreted as ‘basal Ypresian, ~54 Myr’ [26] . Thus, most of the mammalian fossils, including Cambaytherium , appear to be approximately 1.0–1.5 Myr younger than the Palaeocene–Eocene thermal maximum. On the basis of new discoveries presented here, cambaytheres are identified as the sister group of Perissodactyla, showing a mosaic of anatomical traits typical of perissodactyls together with primitive retentions otherwise seen in ‘condylarths’ but not in any known perissodactyls. Discovery of these fossils in the early Eocene of Gujarat suggests that Perissodactyla may have originated on India before its collision with Asia. Fossil sample We document a large, new sample of Cambaytherium thewissi from the early Eocene (early Ypresian) Cambay Shale Formation at Vastan and Mangrol lignite mines in Gujarat, India. It consists of more than 120 dental and gnathic specimens, including two skulls, and nearly 100 postcranial bones ( Figs 1 , 2 , 3 , 4b and 5b,e ; Supplementary Note 1 ), which provide substantial new anatomical data indicating that Cambaytherium is morphologically intermediate between ‘condylarths’ and Perissodactyla. Dental and postcranial regressions developed from extant ungulates [32] indicate that C. thewissi had a body mass of ~20–35 kg, about the size of the peccary Tayassu pecari . 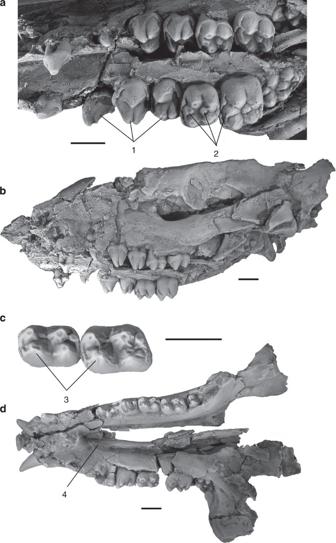Figure 1: Skull and mandible ofCambaytherium thewissi. (a,b) Skull (GU 402) in lateral view and (c,d) mandible (GU 403) in dorsal (occlusal) view.c, right M1–2, enlarged. Key features include: 1, non-molariform premolars; 2, bunodont molars with large conules; 3, twinned molar metaconids; 4, fused symphysis. Scale bars, 1 cm. Figure 1: Skull and mandible of Cambaytherium thewissi . ( a , b ) Skull (GU 402) in lateral view and ( c , d ) mandible (GU 403) in dorsal (occlusal) view. c , right M 1–2 , enlarged. Key features include: 1, non-molariform premolars; 2, bunodont molars with large conules; 3, twinned molar metaconids; 4, fused symphysis. Scale bars, 1 cm. 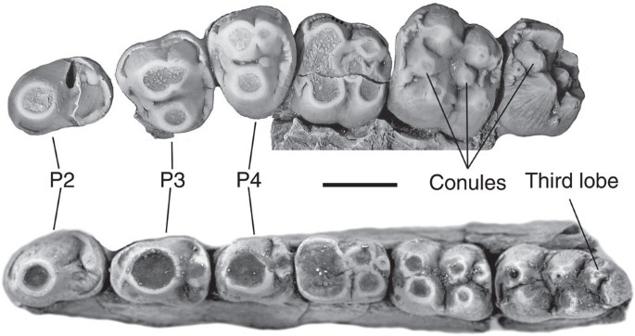Figure 2: Upper and lower cheek teeth of matureCambaytherium thewissi. (a) Left P2–M3(GU 404). (b) Right P2–M3(GU 7004). Note bunodonty, heavy wear, large molar conules, P2–4simple and P2–3larger than P4, M3with large third lobe. Scale bar, 1 cm. Full size image Figure 2: Upper and lower cheek teeth of mature Cambaytherium thewissi . ( a ) Left P 2 –M 3 (GU 404). ( b ) Right P 2 –M 3 (GU 7004). Note bunodonty, heavy wear, large molar conules, P 2–4 simple and P 2–3 larger than P 4 , M 3 with large third lobe. Scale bar, 1 cm. 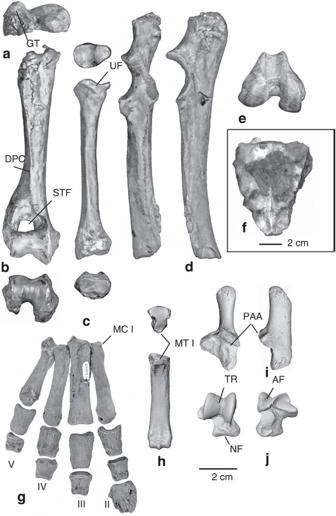Figure 3: Postcranial bones ofCambaytherium thewissiand,Kalitheriumsp. (a) Proximal right humerus (medial view, GU 809). (b) Distal right humerus (anterior and distal views, GU 834). (c) Right radius (proximal, posterior, distal views, GU 274). (d) Right ulna (anterior and medial views, GU 7005). (e) Distal right femur (GU 198). (f) Sacrum (Kalitherium?, GU 8001). (g) Reconstructed right manus (dorsal view of MC II–V and phalanges, positions uncertain; multiple individuals). (h) Left MT III (proximal and posterior views, GU 735). (i) Left calcaneus (dorsal and lateral views, WIF/A-1190). (j) Right astragalus (dorsal and ventral views, GU 780). AF, astragalar foramen; DPC, deltopectoral crest; GT, greater tuberosity; MC I, facet on MC II for first metacarpal; MT I, facet on MT III for vestigial MT I; NF, navicular facet; PAA, posterior astragalar articulation; STF, supratrochlear foramen; TR, trochlea; UF, ulnar facet. Scale bars, 2 cm. Full size image Figure 3: Postcranial bones of Cambaytherium thewissi and, Kalitherium sp. ( a ) Proximal right humerus (medial view, GU 809). ( b ) Distal right humerus (anterior and distal views, GU 834). ( c ) Right radius (proximal, posterior, distal views, GU 274). ( d ) Right ulna (anterior and medial views, GU 7005). ( e ) Distal right femur (GU 198). ( f ) Sacrum ( Kalitherium ?, GU 8001). ( g ) Reconstructed right manus (dorsal view of MC II–V and phalanges, positions uncertain; multiple individuals). ( h ) Left MT III (proximal and posterior views, GU 735). ( i ) Left calcaneus (dorsal and lateral views, WIF/A-1190). ( j ) Right astragalus (dorsal and ventral views, GU 780). AF, astragalar foramen; DPC, deltopectoral crest; GT, greater tuberosity; MC I, facet on MC II for first metacarpal; MT I, facet on MT III for vestigial MT I; NF, navicular facet; PAA, posterior astragalar articulation; STF, supratrochlear foramen; TR, trochlea; UF, ulnar facet. Scale bars, 2 cm. 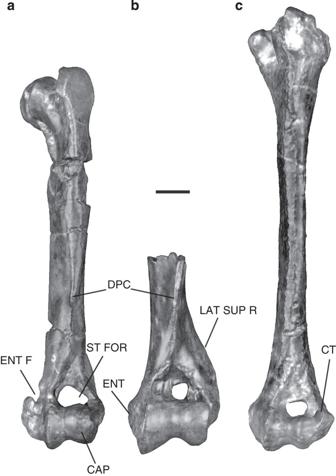Figure 4: Left humeri in anterior view. (a)Phenacodus vortmani(USGS 7159). (b)Cambaytherium thewissi(GU 7006). (c)Homogalax protapirinus(USGS 25032), to same scale. CAP, capitulum; CT, capitular tail; DPC, deltopectoral crest; ENT, entepicondyle; ENT F, entepicondylar foramen; LAT SUP R, lateral supracondylar ridge; ST FOR, supratrochlear foramen. Entepicondylar foramen (Phenacodusonly), distally extensive deltopectoral crest, rounded capitulum and prominent lateral supracondylar ridge are primitive traits.Cambaytheriumand the primitive perissodactylHomogalaxare derived in losing the entepicondylar foramen, andHomogalaxis further derived in being more elongate, with reduced deltopectoral and lateral supracondylar crests, and a conspicuous capitular tail. Scale bar, 1 cm. Full size image Figure 4: Left humeri in anterior view. ( a ) Phenacodus vortmani (USGS 7159). ( b ) Cambaytherium thewissi (GU 7006). ( c ) Homogalax protapirinus (USGS 25032), to same scale. CAP, capitulum; CT, capitular tail; DPC, deltopectoral crest; ENT, entepicondyle; ENT F, entepicondylar foramen; LAT SUP R, lateral supracondylar ridge; ST FOR, supratrochlear foramen. Entepicondylar foramen ( Phenacodus only), distally extensive deltopectoral crest, rounded capitulum and prominent lateral supracondylar ridge are primitive traits. Cambaytherium and the primitive perissodactyl Homogalax are derived in losing the entepicondylar foramen, and Homogalax is further derived in being more elongate, with reduced deltopectoral and lateral supracondylar crests, and a conspicuous capitular tail. Scale bar, 1 cm. 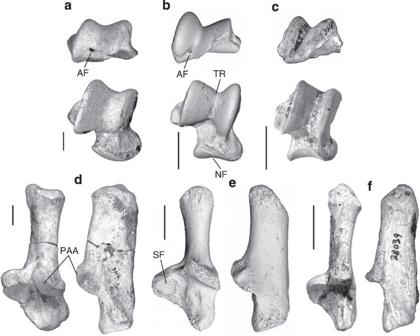Figure 5: Right astragali and left calcanei ofCambaytheriumand comparative taxa. (a–c) astragali in posterior view (above, dorsal at top) and dorsal view; (d–f) calcanei in dorsal and lateral views. (a,d)Phenacodus primaevus(USGS 7146). (b,e)Cambaytherium thewissi(b, GU 780;e, WIF/A-1190). (c,f) cf.Arenahippussp. (c, USGS 25157;f, USGS 38039). Each series scaled to same length; scale bars, 1 cm.Cambaytheriumshares several primitive traits withPhenacodus(not found in primitive perissodactyls), including a dorsal astragalar foramen, wide astragalar trochlea and longer neck, robust calcaneus with wider ectal and sustentacular facets and a rounded ectal facet. Derived traits shared with perissodactyls include a deeper astragalar trochlea and concave navicular facet, though the latter is shallower than in perissodactyls. AF, astragalar foramen; NF, navicular facet; PAA, posterior astragalar articulation; SF, sustentacular facet; TR, trochlea. Full size image Figure 5: Right astragali and left calcanei of Cambaytherium and comparative taxa. ( a – c ) astragali in posterior view (above, dorsal at top) and dorsal view; ( d – f ) calcanei in dorsal and lateral views. ( a , d ) Phenacodus primaevus (USGS 7146). ( b , e ) Cambaytherium thewissi ( b , GU 780; e , WIF/A-1190). ( c , f ) cf. Arenahippus sp. ( c , USGS 25157; f , USGS 38039). Each series scaled to same length; scale bars, 1 cm. Cambaytherium shares several primitive traits with Phenacodus (not found in primitive perissodactyls), including a dorsal astragalar foramen, wide astragalar trochlea and longer neck, robust calcaneus with wider ectal and sustentacular facets and a rounded ectal facet. Derived traits shared with perissodactyls include a deeper astragalar trochlea and concave navicular facet, though the latter is shallower than in perissodactyls. AF, astragalar foramen; NF, navicular facet; PAA, posterior astragalar articulation; SF, sustentacular facet; TR, trochlea. Full size image Summary tooth measurements and statistics are presented in Supplementary Tables 1 and 2 . Measurements of Cambaytherium teeth are normally distributed (41 of 44 dimensions, based on the Shapiro–Wilk statistic) and have low coefficients of variation ( ≪ 10), implying that the sample represents a single species. Although there is considerable variation in occlusal morphology, especially regarding accessory cusps on both premolars and molars (see Supplementary Discussion ), consistent groups are not evident. Consequently, we interpret this as intraspecific variation and refer the sample to the type species of Cambaytherium , C. thewissi Bajpai et al. [16] , which is the only valid species from the Cambay Shale Formation. Evidence will be provided elsewhere to support synonymy of C. bidens and C. minor with C. thewissi . Comparative anatomy Most anatomical features of Cambaytherium (see Supplementary Discussion ) closely resemble those of basal perissodactyls such as Homogalax , Arenahippus and Protorohippus (the latter two genera formerly included in Hyracotherium [33] ), as described below. Many features, however, are more plesiomorphic, often recalling the traits of primitive ungulates like phenacodontids. Cambaytherium shares some traits, related to incipient cursorial adaptation, with both groups. Among them are mesaxonic foot symmetry and hoof-like terminal phalanges, a large third trochanter on the femur, and prominent greater tuberosity on the humerus and greater trochanter on the femur, though the last two features are less developed than in perissodactyls and closer to the condition in phenacodontids ( Fig. 3a ). The distal humeral articulation is narrow and deep and has a large supratrochlear foramen (to accommodate the ulnar anconeal process), which would have enabled greater extension of the forearm, presumably resulting in increased stride length [34] . The radius is positioned anterior to the ulna and articulates with both capitulum and trochlea at an uneven joint that allowed little or no rotation. Derived craniodental traits that unequivocally link Cambaytherium with Perissodactyla include a transverse nasofrontal suture, fused mandibular symphysis, twinned lower molar metaconids and a well-developed third lobe on the last lower molar ( Figs 1 and 2 ). In the postcranial skeleton, Cambaytherium and perissodactyls share an alternating tarsus in which the astragalus is deeply grooved and has a wide, saddle-shaped (concave) articulation for the navicular (the classic perissodactyl synapomorphy [3] ) and a narrow articulation with the cuboid ( Figs 3 and 5 ). Articular facets on Mt III ( Fig. 3h ) indicate that the entocuneiform was rotated posterior to the second metatarsal (Mt II) so that the vestigial Mt I articulated with both the entocuneiform and Mt III, a condition unique to perissodactyls [3] . In the forelimb, the humerus has moderately reduced epicondyles and lacks an entepicondylar foramen. The humeral trochlea is relatively wider and the capitulum narrower than in phenacodontids, closely approaching the perissodactyl condition. In combination, these features occur only in Perissodactyla. Together with these unmistakable perissodactyl traits, Cambaytherium retains many plesiomorphic features lost in perissodactyls but often present in phenacodontid condylarths. In particular, the cheek teeth are bunodont with well-developed conules on the upper molars, and they lack any hint of bilophodonty (which characterizes primitive perissodactyls as well as basal proboscideans) except when heavily worn ( Figs 1 and 2 ). The prominent conules are larger than those in even the most primitive perissodactyls. This may be a uniquely derived trait of cambaytheres and anthracobunids; and it contrasts with basal proboscideans, which lack molar conules [21] . The premolars exhibit little molarization compared with those of early perissodactyls. The skeleton is relatively robust and less adapted for cursorial locomotion than that of basal perissodactyls. In contrast to perissodactyls, the humerus has a moderately developed lateral supracondylar ridge, and the deltopectoral crest is distinct and almost reaches the distal articulation as in phenacodontids. The epicondyles, though reduced, are larger than in most perissodactyls; and the radial articulation lacks the lateral extension (capitular tail) found in all basal perissodactyls ( Fig. 4 ). Most tarsal elements are shorter and wider than in perissodactyls. The calcaneus has a rounded posterior astragalar articulation (unlike the interlocking angular ectal facet of most primitive perissodactyls); and the astragalus has a shorter and wider trochlea, a dorsal astragalar foramen or remnant thereof (unknown in any perissodactyl), a longer neck and a wider cuboid facet ( Fig. 5 ). Five metapodials were present on both manus and pes ( Fig. 3 ), as in phenacodontids. On the basis of the extent and orientation of articular facets, the first metapodial was probably vestigial and thus more reduced than in phenacodontids. The other metapodials were short, stout and flat, unlike the more slender and elongate metapodials of primitive perissodactyls. Cambaytherium is more primitive than any perissodactyl in having evidence of Mc I, and it is more primitive than any perissodactyl with the possible exception of Arenahippus in possessing at least a vestigial Mt V. Overall, the anatomy of Cambaytherium indicates a more omnivorous diet and less cursorially adapted skeleton than in early perissodactyls. Phylogenetic relationships To investigate the phylogenetic position of cambaytheres, we conducted a parsimony analysis of 52 taxa and 208 morphological characters (see Supplementary Notes 2 and 3 ). Besides Cambaytherium and Nakusia , taxa included representatives of anthracobunids, afrotheres and perissodactyls, as well as other ungulates implicated in perissodactyl origins, to test hypotheses of relationships between cambaytheres and these groups. The analysis recovered nine shortest trees of 1,166 steps. In these nine shortest trees, cambaytheres and anthracobunids were always united with perissodactyls to the exclusion of afrotheres, artiodactyls and phenacodontids, with cambaytheres always recovered at the base of the perissodactyl stem ( Fig. 6 ). These results support the hypothesis that cambaytheres are basal members of the clade including perissodactyls and are remnants on the Indian subcontinent of the earliest diversification of this clade. The results also support the identification of anthracobunids as closely related to Perissodactyla rather than Proboscidea. In fact, anthracobunids nest well within Perissodactyla. We suspect, however, that anthracobunids, which are currently known only from teeth, might actually be more closely related to cambaytheres, given their similarities [17] . (See Supplementary Discussion for further consideration of other aspects of the topology recovered.) Discovery of material from the cranial and postcranial skeleton of anthracobunids will provide the best test of this hypothesis. 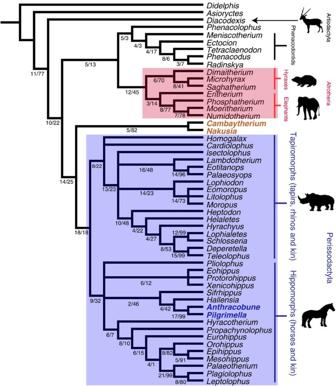Figure 6: Strict consensus of nine shortest trees recovered from parsimony analysis. Shaded boxes indicate Perissodactyla (blue) and Afrotheria (red). Bold taxa indicate cambaytheres (brown) and anthracobunids (blue). Numbers along the branches indicate support values, with Bremer decay index followed by bootstrap support. Figure 6: Strict consensus of nine shortest trees recovered from parsimony analysis. Shaded boxes indicate Perissodactyla (blue) and Afrotheria (red). Bold taxa indicate cambaytheres (brown) and anthracobunids (blue). Numbers along the branches indicate support values, with Bremer decay index followed by bootstrap support. Full size image Although this analysis recovered the shortest trees, it does not support Laurasiatheria (including Perissodactyla and Artiodactyla) exclusive of Afrotheria, which is supported by molecular and combined analyses [7] , [8] , [10] . Therefore, we ran additional phylogenetic analyses using topological constraints—specifically, constraining Artiodactyla and Perissodactyla to be united in Laurasiatheria, and Anthracobunidae to be united with Proboscidea, as previously proposed [23] , [24] , [35] (see Methods and Supplementary Table 3 )—to see if these changes affected the position of cambaytheres. Both analyses also placed cambaytheres at the base of Perissodactyla, either as the sister taxon of Perissodactyla (anthracobunid-Proboscidea constraint) or as the sister taxon of a clade consisting of Anthracobunidae+Perissodactyla (when perissodactyls and artiodactyls were constrained to be closer to each other than to afrotheres). The latter constraint resulted in 49 shortest trees of 1,169 steps, the strict consensus of which is shown in Supplementary Fig. 1 . Anthracobunids and cambaytheres appear as successive sister taxa to perissodactyls, with cambaytheres more basal. The analysis constraining anthracobunids and proboscideans to be monophyletic resulted in four trees of 1,173 steps. The strict consensus of these trees ( Supplementary Fig. 2 ) also places cambaytheres as the sister taxon of perissodactyls. Thus, in all of these analyses, cambaytheres are at the base of the perissodactyl clade. An analysis constraining a monophyletic grouping of cambaytheres, anthracobunids and afrotheres increased the length of the most parsimonious trees to 1,174 steps ( Supplementary Fig. 4 ). The Templeton test [36] did not recover a significant difference in the length of the competing phylogenetic hypotheses ( P =0.318–0.410). Nevertheless, we argue that the cambaythere–perissodactyl clade, as recovered in most of our analyses, is much more probable based on the anatomical features described above, many of which closely approximate those of Perissodactyla and conflict with those of basal afrotheres. Hooker [3] concluded that Asia was the most likely center of origin for Perissodactyla. The presence of cambaytheres uniquely in Indo–Pakistan supports this hypothesis and further suggests what is now southern Asia as the geographic source. The precise pathway of the Indian Plate during its northward drift after separating from Madagascar in the Late Cretaceous, as well as potential continental connections and the timing of collision with Asia, are poorly understood. If current models suggesting isolation of India during the Palaeocene and initiation of collision at 50 Ma or later [37] , [38] , [39] are correct, then it is very unlikely that Cambaytherium reached India from the Asian mainland. European affinities of much of the Vastan mammal assemblage [18] , [19] , [40] , [41] instead support models indicating island arcs or potential land connections with Afro–Arabia during northward drift [7] , [23] , [42] . These models show Gujarat 5–10° south of the equator when the Cambay Shale was deposited [27] , [37] , [38] , [43] ( Fig. 7 ), which would put it closer to Afro–Arabia than to Asia. This suggests that stem taxa leading to perissodactyls could have dispersed to India from Afro–Arabia or a contiguous area, perhaps early in the Palaeocene, and given rise to Perissodactyla before India’s contact with Asia. Palaeocene fossils from India, currently unknown, could provide direct evidence to test this hypothesis. 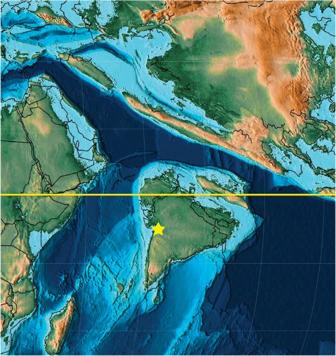Figure 7: Paleomap showing location of Vastan mine (star). Map shows the position of India at the beginning of the Eocene, ~1 Myr before theCambaytheriumfossils; equator highlighted. Figure reproduced with permission from Scotese43. Figure 7: Paleomap showing location of Vastan mine (star). Map shows the position of India at the beginning of the Eocene, ~1 Myr before the Cambaytherium fossils; equator highlighted. Figure reproduced with permission from Scotese [43] . Full size image Sample Fossils are catalogued in the collections of Garhwal University (GU), Srinagar and Wadia Institute of Himalayan Geology (WIF), Dehradun, both in Uttarakhand, India. Comparative specimens illustrated are from the collection of the U.S. Geological Survey (USGS), Denver, which was transferred to the Department of Paleobiology at the National Museum of Natural History, Smithsonian Institution, Washington, D.C. Images Images of fossils were produced either by conventional digital photography (with some specimens lightened with ammonium chloride), laser scanning or microcomputed tomography. Phylogenetic methods A matrix of 208 characters was scored for 52 taxa (see Supplementary Notes 2 and 3 ) to investigate the phylogenetic position of cambaytheres. The character–taxon matrix is available on MorphoBank (Project 1207). Taxa included cambaytheres; the anthracobunids Anthracobune and Pilgrimella ; representatives of perissodactyls, hyracoids, proboscideans, phenacodontids and artiodactyls; the possible perissodactyl relative Radinskya ; the phenacolophid Phenacolophus ; the Cretaceous eutherian Asioryctes ; and the didelphid marsupial Didelphis . Because molecular studies indicate that perissodactyls and afrotheres share a distant common ancestry among placentals, we included a Cretaceous eutherian and a marsupial as outgroups. Characters were compiled from published sources [4] , [5] , [11] , [44] , [45] . In many cases, these characters were modified and new characters and character states were developed. In compiling characters, we made changes to avoid redundancy and to ensure character independence, for example, by comparing the distributions of characters of occluding upper and lower teeth that might be functionally related. Taxa were scored based on personal observation of specimens or casts whenever possible, and in other cases were based on the literature. Parsimony analysis was conducted in PAUP* [46] using heuristic searches, and in TNT [47] using ratchet and TBR, set to recover the shortest tree in 100 different iterations. Didelphis was formally designated as the outgroup for rooting purposes. Bootstrap and Bremer decay analyses were performed in TNT. Gingerich et al. [23] described an isolated astragalus that they attributed to Anthracobune pinfoldi . This astragalus displays none of the perissodactyl-like features of that of Cambaytherium . Its morphology was used as evidence to support a close relationship between anthracobunids and proboscideans [23] . We included data from this astragalus in the analysis reported above; nevertheless, the results support inclusion of anthracobunids in Perissodactyla and do not support a close relationship to Proboscidea. Because this astragalus is not associated with teeth, however, there is reason to question its attribution to Anthracobune . We therefore performed a second analysis where we deleted scores for Anthracobune based on this astragalus, to test the effect of excluding data from this specimen. The resulting analysis produced 29 shortest trees of 1,159 steps ( Supplementary Fig. 3, Supplementary Table 3 ). The results are concordant with the main points of the first analysis, specifically the relationship of cambaytheres and anthracobunids to perissodactyls. The main differences in the results are that anthracobunids are sometimes not nested within Perissodactyla but are recovered as its sister taxon, and Radinskya sometimes comes out as sister taxon to the perissodactyl–anthracobunid clade. Thus, despite the alleged similarities between the supposed Anthracobune astragalus and that of proboscideans, we find no support for allying anthracobunids with proboscideans. Our results support perissodactyl affinities for anthracobunids, regardless of whether or not data from the putative astragalus of Anthracobune are included. Similarly, the phylogenetic position of cambaytheres did not change whether or not these astragalar data were included; therefore, we included them in subsequent analyses described below. We conducted three additional analyses using topological constraints in PAUP* [46] . One of these was to assess the two competing phylogenetic hypotheses of cambaythere relationships—either affinities with Perissodactyla or affinities with Afrotheria (specifically Proboscidea)—by determining the cost in tree length of uniting cambaytheres and anthracobunids with afrotheres. A Templeton test [36] was run to compare the differences in tree length statistically. The other two constrained analyses examined the effect on cambaythere phylogeny of enforcing constraints reflecting other reported relationships. How to cite this article : Rose, K. D. et al. Early Eocene fossils suggest that the mammalian order Perissodactyla originated in India. Nat. Commun. 5:5570 doi: 10.1038/ncomms6570 (2014).